RNA-binding proteins regulate the expression of the immune activating ligand MICB The recognition of stress-induced ligands by the activating receptor NKG2D expressed on cytotoxic lymphocytes is crucial for the prevention and containment of various diseases and is also one of the best-studied examples of how danger is sensed by the immune system. Still, however, the mechanisms leading to the expression of the NKG2D ligands are far from being completely understood. Here, we use an unbiased and systematic RNA pull-down approach combined with mass spectrometry to identify six RNA-binding proteins (RBPs) that bind and regulate the expression of MICB, one of the major stress-induced ligands of NKG2D. We further demonstrate that at least two of the identified RBPs function during genotoxic stress. Our data provide insights into stress recognition and hopefully open new therapeutic venues. Natural Killer (NK) cells are innate lymphocytes that are able to discriminate between self and non/altered-self to eliminate virally infected, transformed and damaged cells [1] , [2] , [3] . In addition, NK cells regulate and support developmental processes such as fetal growth during pregnancy [4] . Both, the cytotoxic and regulatory activities of NK cells are controlled by germline-encoded inhibitory and activating receptors [5] , [6] . The inhibitory receptors are expressed stochastically and the number of inhibitory receptors expressed on a given NK cell is correlated with the potency of that specific cell [7] , [8] , a process termed licensing or arming/disarming [9] . The main inhibitory ligands recognized by the inhibitory NK receptors are self-HLA class I proteins [6] , which are expressed by all nucleated cells. In contrast, the activating receptors are expressed by most of the NK cell population and the ligands recognized by these receptors are more diverse in identity and in their expression pattern [5] . The activating ligands can be of self or of non-self origin, and can be either expressed ubiquitously or upregulated following various insults [5] . Of the activating NK cell receptors, NKG2D (which is expressed also by some T-cell subsets) is characterized by binding to ligands that are stress induced [10] . The expression of the stress-induced ligands is induced in various conditions such as viral infection, cell transformation, inflammation, heat shock, DNA damage and following treatment with histone deacetylase inhibitors [2] , [10] , [11] , [12] , [13] , [14] . Humans possess two families of stress-induced NKG2D ligand genes: the human-specific MHC class I-related chain (MIC) gene family (MICA and MICB) and the UL16-binding proteins (ULBP) gene family (ULBP1-6). Many mammals encode genes of the ULBP family only, but lack the MIC family. Specifically, rodents such as mice and rats lack the MIC family of ligands [15] , [16] , indicating that the regulation and recognition of stress by human immune cells is substantially different from that of mice. The mechanisms leading to the expression of the NKG2D ligands are far from being understood. Out of the eight human NKG2D ligands, the regulation of MICA and MICB expression is best studied so far, and it seems as if MICB and MICA are generally regulated by common regulatory mechanisms. At the transcriptional level, the promoter regions of MICA and MICB were characterized and both include heat shock protein-binding elements [17] . At the post-transcriptional level, we have previously identified seven cellular microRNAs (miRNAs) that regulate both MICA and MICB [18] , and three additional miRNAs that regulate only MICB [19] , [20] . Some of these miRNAs such as the miR-17-92 cluster and miR-10b are known oncomiRs or metastamiRs, playing a crucial role in cell transformation or tumour progression. Gene expression is tightly controlled and fine-tuned not only by miRNAs but also by RNA-binding proteins (RBPs) [21] . Soon after transcription initiation, RBPs coat the newly synthesized RNA molecule and are involved in every aspect of RNA biology: transcription, pre-messenger RNA (mRNA) splicing, polyadenylation, RNA modification, transport, localization, translation and turnover [22] , [23] , [24] , [25] . Thus, the function of RBPs is essential for proper gene expression, and their dysfunction can lead to aberrant cellular properties and diseases such as cancer, neurodegenerative, autoimmunity and developmental defects [26] . In the current study, we focused on the RBP-mediated post-transcriptional regulation of the human-specific MIC family. We have identified six RBPs that specifically bind to the 3′UTR of MICB and control its expression. Importantly, we show the function of two RBPs, FUBP3 and HuR during genotoxic stress and their effect on NK cells recognition and elimination of damaged cells. RBPs differentially bind the 3′UTRs of MICA and MICB It is unknown whether RBPs regulate the expression of the human-specific genes, MICA or MICB . To identify RBPs that might bind to the 3′UTR of MICA or MICB, we applied an RNA-affinity purification (RNA-AP) method combined with a mass spectrometry (MS) analysis [27] . The RNA-AP was performed with cytoplasmic extracts, hence excluding most nuclear proteins. We concentrated on studying cytoplasmic proteins as they control localization, stability and translation of transcripts [21] , [22] , [24] . The 3′UTRs of MICA, MICB and control UTRs (listed below) were cloned into pBSII and were in vitro transcribed in the presence of biotinylated-UTP. For each 3′UTR (MICA or MICB), two control UTRs were used: (I) an antisense orientation of the specific UTR (MICA-AS/MICB-AS) and (II) 3′UTR of a different gene that is similar in length and with a similar nucleotide composition (Ctrl-A/Ctrl-B). In addition, to estimate background protein binding, we also purified proteins using unlabelled RNAs (un-MICA/un-MICB) and using only streptavidin beads (BG) without an RNA molecule. Next, cytoplasmic extract of RKO cells was incubated with the various RNAs, precipitated with streptavidin beads and separated on an SDS gel ( Fig. 1 ). The specific bands obtained were precipitated only with the 3′UTR of MICB and not with the 3′UTR of MICA. To validate these results, we repeated the RNA-AP in another cell line, HEK293T, and obtained similar results ( Supplementary Fig. 1 ). To identify the RBPs that were precipitated specifically with the 3′UTR of MICB, we excised protein bands that were either selectively precipitated or showed increased intensity when precipitated with the 3′UTR of MICB in both cell lines (RKO and HEK293T). Thus, proteins that were only precipitated in RKO cells (for example, the proteins found between 34 kDa and 43 kDa, Fig. 1 ), were not considered because they were also found in the ‘AS’ and in the ‘Ctrl-B’ precipitations of the HEK293T cells ( Supplementary Fig.1 ). Band number 2 is an exception as it appears only in the RKO cells and not in 293T cells ( Fig. 1 and Supplementary Fig. 1 ). We also excised this band because it was specifically precipitated with the 3′UTR of MICB in RKO cells. 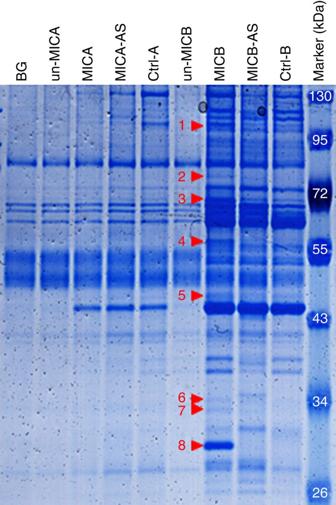Figure 1: RBP precipitation by the 3′UTR of MICB. Coomassie staining of RBPs precipitated from cytoplasmic extracts of RKO cells via RNA-AP. The specific bands that were cut and sent for MS analysis are numbered and marked by red arrowheads. BG-background, stands for purification in the presence of streptavidin beads only (without a labelled RNA). Un-MICA/un-MICB stands for the 3′UTR of either MICA or MICB, which was not labelled with biotinylated UTPs. MICA/MICB stands for the 3′UTR of either MICA or MICB labelled with biotinylated UTPs. AS stands for antisense 3′UTR. Ctrl-A is the 3′UTR of TAF6. Ctrl-B is the 3′UTR of CASQ2. Figure 1: RBP precipitation by the 3′UTR of MICB. Coomassie staining of RBPs precipitated from cytoplasmic extracts of RKO cells via RNA-AP. The specific bands that were cut and sent for MS analysis are numbered and marked by red arrowheads. BG-background, stands for purification in the presence of streptavidin beads only (without a labelled RNA). Un-MICA/un-MICB stands for the 3′UTR of either MICA or MICB, which was not labelled with biotinylated UTPs. MICA/MICB stands for the 3′UTR of either MICA or MICB labelled with biotinylated UTPs. AS stands for antisense 3′UTR. Ctrl-A is the 3′UTR of TAF6. Ctrl-B is the 3′UTR of CASQ2. Full size image We were also interested to see the types of proteins that were precipitated with all of the UTRs. Thus we excised protein band number 3, which was precipitated both with the 3′UTR of MICB and with the control UTRs, both in RKO and in HEK293T cells ( Fig. 1 and Supplementary Fig. 1 ). All protein bands that are marked by red arrowheads in Fig. 1 and in Supplementary Fig. 1 were cut and analysed by MS. We were unable to unequivocally identify the proteins corresponding to bands number 3, 6 and 7. In contrast, the high-ranking proteins that corresponded to bands 1, 2, 4, 5 and 8 were identified and are listed in Table 1 together with their general function and features. Table 1 RBPs—features and function. Full size table Notably, most of the MICB-precipitated proteins bear RNA-recognition motifs ( Table 1 ). FUBP3 and XRN2 are the exceptions that do not encode an RNA-recognition motif and instead have either an hnRNP-K-homology domain or a CCHC-type zinc-finger motif that mediate RNA binding, respectively. Importantly, the identified RBPs have known established functions in the regulation of gene expression and they affect transcription, mRNA stability, translational regulation, mRNA processing and more [28] , [29] , [30] , [31] , [32] , [33] . RBPs interact in vivo with the mRNA of MICB To investigate whether the identified RBPs can interact with MICB in living cells, we used RKO cells (also used in the RNA-AP) whole-cell lysates to perform RNP immunoprecipitation (RIP) experiments according to the protocol described by Peritz T et al . [34] We successfully precipitated FUBP3, HuR, XRN2, CUGBP1, IGF2BP2 and hnRNP-M using specific antibodies. However, we were not able to pull down MATR3 effectively. Specific protein precipitation was verified by western blot (WB, Fig. 2a ). 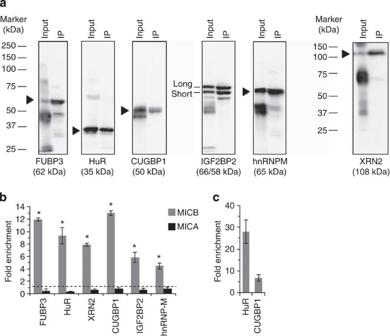Figure 2: The mRNA of MICB endogenously associates with the identified RBPs. RIP analysis was performed with RKO whole-cell lysate. (a) Whole membranes of WB analysis of the immunoprecipitation (IP) of the specific RBPs. Input is total protein input used for the RIP experiment, IP is the sample in which a specific antibody was used (b) Fold enrichment of the mRNAs of MICB (grey) or MICA (black) bound by the specific RBP (xaxis) as assessed by qRT–PCR. Shown are mean±s.e.m. of triplicates. Data are representative of three independent experiments performed. *P<0.003 by paired Student’st-test of all three independent experiments combined. (c) qRT–PCR of known transcripts bound by HuR (β-actin) or CUGBP1 (c-JUN). Shown is mean fold enrichment of the known target relative to total RNA of two independent experiments±s.d. Figure 2: The mRNA of MICB endogenously associates with the identified RBPs. RIP analysis was performed with RKO whole-cell lysate. ( a ) Whole membranes of WB analysis of the immunoprecipitation (IP) of the specific RBPs. Input is total protein input used for the RIP experiment, IP is the sample in which a specific antibody was used ( b ) Fold enrichment of the mRNAs of MICB (grey) or MICA (black) bound by the specific RBP ( x axis) as assessed by qRT–PCR. Shown are mean±s.e.m. of triplicates. Data are representative of three independent experiments performed. * P <0.003 by paired Student’s t -test of all three independent experiments combined. ( c ) qRT–PCR of known transcripts bound by HuR (β-actin) or CUGBP1 (c-JUN). Shown is mean fold enrichment of the known target relative to total RNA of two independent experiments±s.d. Full size image Next, the co-immunoprecipitated RNA bound by the various RBPs was purified and the enrichment levels of MICB and MICA transcripts were assessed by quantitative reverse transcriptase PCR (qRT–PCR) ( Fig. 2b ). As can be seen, MICB, but not MICA mRNA was enriched in all samples ( Fig. 2b ). Known target transcripts of HuR (β-actin) and CUGBP1 (c-JUN) were used as a positive control for the integrity of the assay ( Fig. 2c ). The expression of MICB is regulated by RBPs To investigate whether the MICB mRNA-interacting RBPs can regulate the protein expression of MICB, we transduced RKO cells with lentiviruses encoding short hairpin RNAs (shRNAs) against each RBP. We confirmed the efficiency of the knockdown (KD) by qRT–PCR ( Fig. 3a ) and by WB ( Supplementary Fig. 2a,b ). In addition, we validated the functionality of the KD by assessing the levels of c-JUN, a known target of CUGBP1, and observed a significant increase in c-JUN expression due to CUGBP1 depletion ( Supplementary Fig. 2c ). Subsequently, we analysed the expression of MICB on RKO cells by fluorescence-activated cell sorting (FACS) ( Fig. 3b , quantified in Fig. 3c ). Interestingly, the KD of FUBP3, HuR, XRN2, MATR3 and CUGBP1 resulted in the increased expression of MICB, suggesting that these RBPs negatively regulate MICB expression. We therefore referred to them as negative regulators ( Fig. 3b,c ). Depletion of IGF2BP2 led to reduced expression of MICB, suggesting that it positively regulated MICB (positive regulator, Fig. 3b,c ). Although hnRNP-M binds the MICB mRNA ( Fig. 2 ), the KD of hnRNP-M had no effect (referred as non-regulator), but this might be because of the KD efficiency ( Fig. 3a and Supplementary Fig. 2a,b ). To further control our experiments, we also knocked down the RBP STAU2 ( Fig. 3a ), which was not highly ranked in the MS analysis of the precipitated MICB proteins, and observed no effect on MICB expression ( Fig. 3b , quantified in Fig. 3c ). We thus used this RBP as a negative control in subsequent analyses. All of the various RBP-shRNAs did not affect the levels of MICA on the cell surface of RKO cells ( Fig. 3d ). To further establish the specificity of the RBPs for the regulation of MICB and not MICA and because RKO cells express low or no MICA, we also assessed the levels of MICA on HEK293T cells that were transduced with shRNAs targeting the various RBPs. As can be seen, the KD of the various RBPs did not affect the expression levels of MICA ( Supplementary Fig. 3a ). 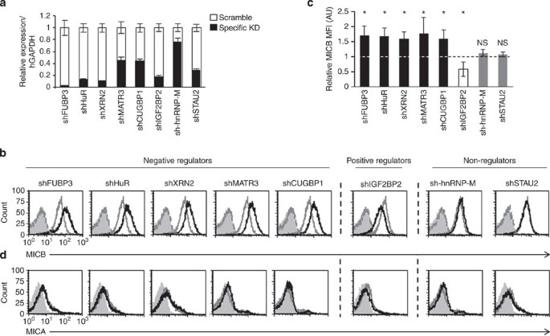Figure 3: Depletion of the identified RBPs alters the surface expression of MICB. (a) Quantitative RT–PCR was performed to validate the KD of the RBPs of interest. Shown is the relative abundance in RKO cells. Relative abundance in cells transduced with a control-shRNA was set as 1. ThehGAPDHgene was used as a reference gene. Shown are mean±s.e.m. of triplicates. Data are representative of three independent experiments. (b) FACS analysis of the expression of MICB on RKO cells transduced with the indicated RBP-shRNAs. The empty black histogram represents the indicated shRNA, the empty grey histogram represents a control-shRNA, the dashed dark grey histogram represents background of the indicated shRNA and the filled grey histogram represents background staining of control-shRNA. Data are representative of six independent experiments. (c) Quantification of the effect of the various RBPs on the levels of MICB expression in RKO cells. Shown is the relative average MFI of MICB±s.d. in six independent experiments calculated relative to the average MFI by Ctrl-shRNA-transduced RKO cells (set as 1). *P<0.009, by paired Student’st-test, NS, not significant. (d) FACS analysis of the expression of MICA on RKO cells transduced with the indicated shRNAs. The empty black histogram represents the indicated shRNA, the empty grey histogram represents a control-shRNA, the dashed dark grey histogram represents background of the indicated shRNA and the filled grey histogram represents background staining of control-shRNA. Data are representative of six independent experiments. Figure 3: Depletion of the identified RBPs alters the surface expression of MICB. ( a ) Quantitative RT–PCR was performed to validate the KD of the RBPs of interest. Shown is the relative abundance in RKO cells. Relative abundance in cells transduced with a control-shRNA was set as 1. The hGAPDH gene was used as a reference gene. Shown are mean±s.e.m. of triplicates. Data are representative of three independent experiments. ( b ) FACS analysis of the expression of MICB on RKO cells transduced with the indicated RBP-shRNAs. The empty black histogram represents the indicated shRNA, the empty grey histogram represents a control-shRNA, the dashed dark grey histogram represents background of the indicated shRNA and the filled grey histogram represents background staining of control-shRNA. Data are representative of six independent experiments. ( c ) Quantification of the effect of the various RBPs on the levels of MICB expression in RKO cells. Shown is the relative average MFI of MICB±s.d. in six independent experiments calculated relative to the average MFI by Ctrl-shRNA-transduced RKO cells (set as 1). * P <0.009, by paired Student’s t -test, NS, not significant. ( d ) FACS analysis of the expression of MICA on RKO cells transduced with the indicated shRNAs. The empty black histogram represents the indicated shRNA, the empty grey histogram represents a control-shRNA, the dashed dark grey histogram represents background of the indicated shRNA and the filled grey histogram represents background staining of control-shRNA. Data are representative of six independent experiments. Full size image We also cloned all of the above-mentioned RBPs into a lentiviral vector that also expressed a green fluorescent protein cassette (reporting for transduction efficiency) ( Fig. 4a ) and transduced RKO cells with the various RBPs. Complementary to the KD data ( Fig. 3 ), overexpression of FUBP3, HuR, XRN2, MATR3 and CUGBP1 led to reduced expression of MICB, while it did not alter the levels of MICA on the transduced RKO cells ( Fig. 4b,c , the changes observed in MICB levels were quantified in Fig. 4d ). Two variants of the positive regulator IGF2BP2 (ref. 35) [35] were cloned; named here IGF2BP2-short and IGF2BP2-long. Interestingly, the expression of IGF2BP2-short but not IIGF2BP2-long resulted in increased cell surface expression of MICB ( Fig. 4b,d ), while both isoforms did not affect the levels of MICA ( Fig. 4c ). Overexpression of hnRNP-M had no effect on the levels of MICB or MICA ( Fig. 4b–d ), supporting the KD results presented in Fig. 3b . To further establish the specificity of the RBPs to MICA and not to MICB, we also assessed the levels of MICA on HEK293T cells (that express high levels of MICA) transduced with the various RBPs. As expected, the overexpression of the various RBPs did not affect the expression levels of MICA ( Supplementary Fig. 3b ). 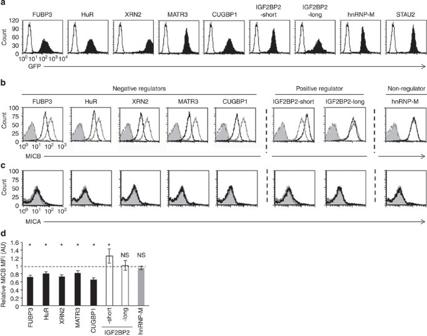Figure 4: Overexpression of the identified RBPs alters the surface expression of MICB. (a) Green fluorescent protein (GFP) levels of RKO cells transduced with the various indicated RBPs. The empty black histogram represents background autofluorescence, the filled black histogram represents GFP expression after transduction. (b,c) FACS analysis of the expression of MICB (b) and of MICA (c) on RKO cells transduced with the indicated RBP. The empty black histogram represents the indicated RBP (gated on GFP+cells), the empty grey histogram represents the control RBP (STAU2). The dashed dark grey histogram represents background of the indicated RBP and the filled grey histogram represents background staining of STAU2 cells. (d) Quantification of the effect of the various RBPs on the levels of MICB in RKO cells. Shown is the relative average MFI of MICB±s.d. from six independent experiments calculated relative to the average MFI by STAU2-transduced RKO cells (set as 1). *P<0.05, by paired Student’st-test, NS, not significant. Figure 4: Overexpression of the identified RBPs alters the surface expression of MICB. ( a ) Green fluorescent protein (GFP) levels of RKO cells transduced with the various indicated RBPs. The empty black histogram represents background autofluorescence, the filled black histogram represents GFP expression after transduction. ( b , c ) FACS analysis of the expression of MICB ( b ) and of MICA ( c ) on RKO cells transduced with the indicated RBP. The empty black histogram represents the indicated RBP (gated on GFP + cells), the empty grey histogram represents the control RBP (STAU2). The dashed dark grey histogram represents background of the indicated RBP and the filled grey histogram represents background staining of STAU2 cells. ( d ) Quantification of the effect of the various RBPs on the levels of MICB in RKO cells. Shown is the relative average MFI of MICB±s.d. from six independent experiments calculated relative to the average MFI by STAU2-transduced RKO cells (set as 1). * P <0.05, by paired Student’s t -test, NS, not significant. Full size image RBP-mediated regulation of MICB affects NK-mediated killing To investigate whether the RBP-dependent modulation of MICB expression was of functional relevance, we performed NK cytotoxicity assays on cells transduced with the various RBP-shRNAs or overexpression constructs. Primary bulk human NK cells were incubated for 5 h with 35 S-methionine-labelled target cells and killing levels were assessed ( Fig. 5 ). The killing of RBP–KD cells was compared with control-shRNA-transduced cells (Ctrl, set to 1, Fig. 5a–c ), while the killing of cells that overexpressed the respective RBPs was compared with STAU2-overexpressing cells ( Fig. 5d–f ); the killing of STAU2-overexpressing cells was set as 1. 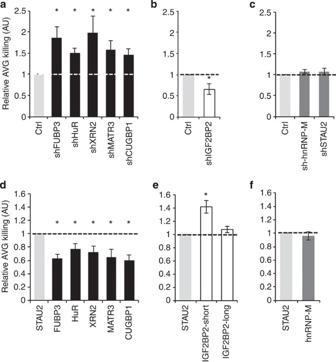Figure 5: Alteration in MICB expression affects killing by NK cells. (a–f) [35S]methionine-labelled cells transduced with the indicated vectors (either shRNA (a–c), or the specific RBP (d–f),xaxis) were incubated for 5 h with bulk primary NK cells, and then killing levels were assessed. Data are the summation total of six independent experiments (by three donors). (a–c) Target cells transduced with a control-shRNA were used as a control and their killing levels were set to 1. Shown is the relative average killing±s.d. of three independent experiments.*P<0.005, by paired Student'st-test. (d–f) Target cells transduced with STAU2 were used as a control and their killing levels were set to 1. Shown is the relative average killing±s.d. of three independent experiments.*P<0.005, by paired Student'st-test. Figure 5: Alteration in MICB expression affects killing by NK cells. ( a – f ) [ 35 S]methionine-labelled cells transduced with the indicated vectors (either shRNA ( a – c ), or the specific RBP ( d – f ), x axis) were incubated for 5 h with bulk primary NK cells, and then killing levels were assessed. Data are the summation total of six independent experiments (by three donors). ( a – c ) Target cells transduced with a control-shRNA were used as a control and their killing levels were set to 1. Shown is the relative average killing±s.d. of three independent experiments. *P <0.005, by paired Student's t -test. ( d – f ) Target cells transduced with STAU2 were used as a control and their killing levels were set to 1. Shown is the relative average killing±s.d. of three independent experiments. *P <0.005, by paired Student's t -test. Full size image In agreement with the results presented above, the elevated MICB expression observed following the KD of FUBP3, HuR, XRN2, MATR3 and CUGBP1 ( Fig. 3b ) resulted in increased killing of these cells by NK cells ( Fig. 5a ), while the opposite effect was observed after overexpression of these RBPs ( Fig. 5d ). In addition, KD of the positive MICB regulator IGF2BP2 reduced NK killing ( Fig. 5b ) and its overexpression increased (short form only) killing of cells ( Fig. 5e ). Finally, in accordance with the FACS data ( Figs 3b , 4b ), no changes in killing levels were observed in cells overexpressing IGF2BP2-long ( Fig. 5e ), nor in cells in which hnRNP-M and STAU2 were depleted or overexpressed ( Fig. 5c,f ). Mechanisms of MICB regulation by RBPs RBPs can influence gene expression by various mechanisms including transcription, mRNA stability and regulation of translation [22] , [36] . To elucidate the mechanism by which the identified MICB-targeting RBPs regulate the expression of MICB, we performed qRT–PCR analysis to monitor the mRNA levels of MICB in the various RBP–KD and RBP-overexpressing cells ( Fig. 6a–f ). In the KD experiments, a control-shRNA (Ctrl) was used. In the overexpression experiments, STAU2 served as a negative control. In agreement with the increased surface expression of MICB ( Fig. 3b ), KD of FUBP3, HuR, XRN2, MATR3 and CUGBP1 led to an increased abundance of the MICB transcript ( Fig. 6a ). Supporting these results, the overexpression of these RBPs led to a reduced mRNA abundance ( Fig. 6b ), consistent with the reduced MICB surface expression ( Fig. 3b ). This suggests that the identified MICB-targeting RBPs might regulate the expression of MICB by regulating the stability and turnover rate of the MICB transcript. 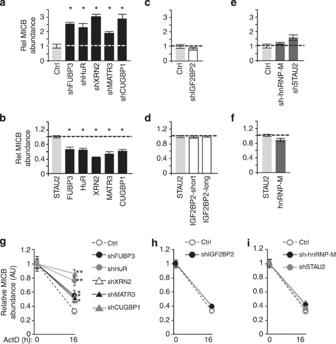Figure 6: Mechanism of RBP-mediated regulation of MICB expression. Relative mRNA abundance of MICB in RKO cells transduced with various shRNAs (a,c,e) or RBPs (b,d,f) was evaluated by qRT–PCR. hGAPDH was used as a reference gene. Shown are mean±s.e.m. of triplicates. Data are representative of three independent experiments. (a,c,e) The abundance of MICB in cells transduced with a control-shRNA was set as 1. (b,d,f) The abundance of MICB in cells transduced with STAU2 was set as 1. *P<0.05, by paired Studentst-test. (g–i) Relative mRNA abundance of MICB in the shRNA-transduced RKO cells treated with ActD was evaluated by qRT–PCR. The abundance of MICB in each RBP–KD cell at time 0 was set as 1. The hGAPDH was used as a reference gene. Shown are mean±s.e.m. of triplicates. Data are representative of three independent experiments. *P<0.02, **P<0.002 by Studentst-test. Figure 6: Mechanism of RBP-mediated regulation of MICB expression. Relative mRNA abundance of MICB in RKO cells transduced with various shRNAs ( a , c , e ) or RBPs ( b , d , f ) was evaluated by qRT–PCR. hGAPDH was used as a reference gene. Shown are mean±s.e.m. of triplicates. Data are representative of three independent experiments. ( a , c , e ) The abundance of MICB in cells transduced with a control-shRNA was set as 1. ( b , d , f ) The abundance of MICB in cells transduced with STAU2 was set as 1. * P <0.05, by paired Students t -test. ( g – i ) Relative mRNA abundance of MICB in the shRNA-transduced RKO cells treated with ActD was evaluated by qRT–PCR. The abundance of MICB in each RBP–KD cell at time 0 was set as 1. The hGAPDH was used as a reference gene. Shown are mean±s.e.m. of triplicates. Data are representative of three independent experiments. * P <0.02, ** P <0.002 by Students t -test. Full size image In contrast, although reduced surface expression of MICB was observed in IGF2BP2-KD cells ( Fig. 3b ), and increased expression of MICB was noticed in cells expressing IGF2BP2-short ( Fig. 4b ), no change was observed in the abundance of the MICB transcript when IGF2BP2 was depleted or overexpressed ( Fig. 6c,d , respectively). This suggests that IGF2BP2 might regulate MICB protein expression by controlling the translation of the MICB mRNA. No change in MICB abundance was observed in hnRNP-M-KD cells or in hnRNP-M-overexpressing cells ( Fig. 6e,f , respectively). Similarly, no significant change was observed in the control STAU2-KD cells ( Fig. 6e ). We also tested the relative abundance of the MICA transcripts and observed no significant change in any of the KD or overexpressing cells ( Supplementary Fig. 4 ). To test whether the increased abundance of MICB mRNA observed in the negative regulator RBPs–KDs was due to increased transcription or changes in the stability of the transcript, we treated the various RBP–KD cells with the transcription inhibitor actinomycin D (ActD). After 16 h, we harvested the cells and analysed the relative abundance of the MICB mRNA. We observed a higher MICB mRNA level after depletion of all negative regulators ( Fig. 6g ). These data suggest that these RBPs post transcriptionally regulate MICB expression by increasing the rate of MICB mRNA decay. Depletion of IGF2BP2, hnRNP-M or STAU2 had no effect on MICB mRNA stability ( Fig. 6h,i ). Putative-binding regions of MICB-regulating RBPs Next, we wanted to identify the regulatory elements in the 3′UTR of MICB that were recognized by the identified RBPs. Since not all of the identified RBPs have known binding sequences ( Table 1 ), we analysed the sequence of the 3′UTR of MICB for the reported binding sites, which are marked in Fig. 7a : AU-rich elements (HuR) [37] ; WWCUUD (MATR3) [38] ; GU-rich elements (CUGBP1) [39] ; and CAUH [40] or the MAWWMA [38] consensus sequences of IGF2BP2. Although no MICA-specific RBPs were precipitated with the 3′UTR of MICA, we analysed the sequence of the 3′UTR of MICA for possible RBP-binding sequences. In agreement with the aforementioned results, of all the known RBP consensus sequences found in the 3′UTR of MICB ( Table 1 ), only a single AU-rich element was found in the 3′UTR of MICA ( Supplementary Fig. 5 ). 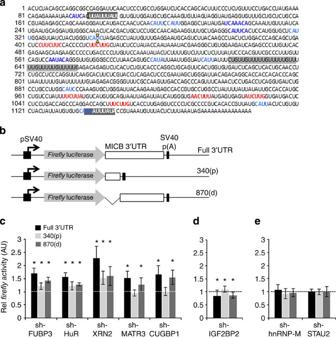Figure 7: Binding regions of the MICB-targeting RBPs in the 3′UTR of MICB. (a) The sequence of the 3′UTR of MICB. Highlighted are potential RBP-binding elements. AU-rich elements (possible HuR-binding regions) are highlighted in dark grey and white letters. A GU-rich element (possible CUGBP1-binding region) is highlighted in dark grey. MATR3 consensus-binding sequences are marked in red. IGF2BP2 consensus binding sequences are marked in blue. The XbaI restriction site was used to generate two UTR fragments, and is marked by two yellow arrows. (b) Schematic description of theFireflyluciferase constructs used. An SV40 promoter (black arrow) drives the expression of theFireflyluciferase (grey arrow), which is fused either to the full-length 3′UTR of MICB (‘full 3′UTR’, top), to the proximal 340 bp of the 3′UTR (‘340(p)’, middle), or to the distal 870 bp of the 3′UTR (‘870(d)’, bottom). (c–e) The threeFireflyreporters were transfected into RKO cells transduced with the various shRNAs (indicated on thexaxis). Forty-eight hours post transfection,Fireflyactivity was measured relative to theRenillaluciferase. TheFirefly/Renillaactivity ratio was normalized to the ratio in the control-shRNA-transduced cells, which was set to 1. Shown is averaged mean±s.d. of combined six independent experiments. *P<0.05, by Student’st-test. White/black line represents the one threshold. Figure 7: Binding regions of the MICB-targeting RBPs in the 3′UTR of MICB. ( a ) The sequence of the 3′UTR of MICB. Highlighted are potential RBP-binding elements. AU-rich elements (possible HuR-binding regions) are highlighted in dark grey and white letters. A GU-rich element (possible CUGBP1-binding region) is highlighted in dark grey. MATR3 consensus-binding sequences are marked in red. IGF2BP2 consensus binding sequences are marked in blue. The XbaI restriction site was used to generate two UTR fragments, and is marked by two yellow arrows. ( b ) Schematic description of the Firefly luciferase constructs used. An SV40 promoter (black arrow) drives the expression of the Firefly luciferase (grey arrow), which is fused either to the full-length 3′UTR of MICB (‘full 3′UTR’, top), to the proximal 340 bp of the 3′UTR (‘340(p)’, middle), or to the distal 870 bp of the 3′UTR (‘870(d)’, bottom). ( c – e ) The three Firefly reporters were transfected into RKO cells transduced with the various shRNAs (indicated on the x axis). Forty-eight hours post transfection, Firefly activity was measured relative to the Renilla luciferase. The Firefly/Renilla activity ratio was normalized to the ratio in the control-shRNA-transduced cells, which was set to 1. Shown is averaged mean±s.d. of combined six independent experiments. * P <0.05, by Student’s t -test. White/black line represents the one threshold. Full size image To evaluate whether the identified sites were indeed bound by the appropriate RBPs, we generated three reporter plasmids (illustrated in Fig. 7b ): (i) a Firefly luciferase fused to the full-length 3′UTR of MICB (named here ‘full 3′UTR’); (ii) a Firefly luciferase fused to the proximal 340 bp fragment of the 3′UTR (named here ‘340(p)’), which was predicted to contain binding sites for HuR and IGF2BP2, and (iii) a Firefly luciferase fused to the distal 870 bp of the 3′UTR of MICB (named here ‘870(d)’), which was predicted to contain binding sites for HuR, MATR3, CUGBP1 and IGF2BP2. The three reporter plasmids were transfected into the various RKO RBP–KD cells, and the activity ratio of Firefly/Renilla luciferases was assessed ( Fig. 7c–e ). In accordance with the FACS data, an increase in the full 3′UTR reporter activity was observed when the reporter was transfected into cells in which the negative regulators of MICB were knocked down ( Fig. 7c ). KD of the positive regulator, IGF2BP2, resulted in a modestly yet significantly reduced reporter activity ( Fig. 7d ) and the KD of hnRNP-M and STAU2 had no effect ( Fig. 7e ). HuR is known to affect mRNA stability by binding to AU-rich elements. Two classical AU-rich elements are present in the 3′UTR of MICB, one in the 340(p) reporter and the other in the 870(d) reporter ( Fig. 7a , white letters and grey highlight). Indeed, in the HuR–KD cells, when either the 340(p) or the 870(d) reporters were transfected, an increased reporter activity was observed. The reporter activity was less than that observed with the full-length 3′UTR ( Fig. 7c ), probably because the number of AU-rich elements might correlate with the efficiency of HuR-mediated regulation [37] . The consensus-binding sequence of MATR3 was only recently identified [38] , and was found to reside solely in the 870(d) reporter ( Fig. 7a , marked in red). Indeed, KD of MATR3 increased the 870(d) reporter activity, but did not affect the activity of the 340(p) reporter ( Fig. 7c ). Similarly, a binding sequence for CUGBP1 was predicted only in the 870(d) reporter ( Fig. 7a , highlighted in grey), and consequently KD of CUGBP1 increased its activity while the activity of the 340(p) reporter remained unaffected ( Fig. 7c ). FUBP3 and XRN2 affected the activity of all reporters (full length and truncated, Fig. 7c ), suggesting that FUBP3 and XRN2 binding sequence/elements might be present in both 3′UTR fragments. Binding sequences for the positive regulator of MICB, IGF2BP2, were present throughout the 3′UTR of MICB ( Fig. 7a , marked in blue). Indeed, KD of IGF2BP2 led to a modest, but statistically significant decrease in both the full 3′UTR reporter and the 870(d) reporter activity ( Fig. 7d ). Surprisingly, a modest, yet statistically significant increase in the activity of the 340(p) reporter was observed ( Fig. 7d ). Finally, KD of hnRNP-M or STAU2, which had no effect on MICB levels ( Fig. 2b ), had also no effect on the reporter activities ( Fig. 7e ). CUGBP1 binds the 3′UTR of MICB at a GU-rich element Next, we wanted to test whether mutating a predicted RBP-binding site in the 3′ UTR of MICB would affect the regulatory activity of this RBP. We chose to focus on CUGBP1, as this is the only RBP that had a single and well defined, predicted binding element in the 3′UTR of MICB ( Fig. 7a ). The predicted binding element of CUGBP1 in the 3′UTR of MICB consists of GU-rich repeats, and indeed in the 3′UTR of MICB, we found five repeats of the 5′-GUUUUUG-3′ heptamer ( Table 1 and Fig. 8a , top). Thus, we generated a mutated 3′UTR in which we changed every third Uracil in this GU-rich element, to a Guanine ( Fig. 8a , bottom, red letters, named GUmut). We fused the GUmut 3′UTR of MICB to a Firefly luciferase reporter and performed dual luciferase assays in RKO cells. The reporter fused to the mutated 3′UTR showed increased activity in comparison with the reporter fused to the wild type (WT) 3′UTR of MICB, suggesting that indeed this element was important for the negative regulation of MICB expression ( Fig. 8b ). 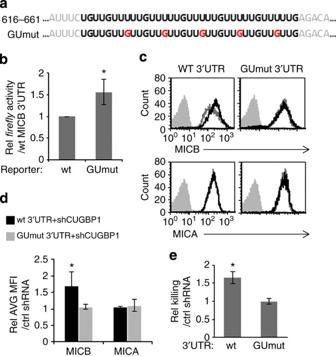Figure 8: CUGBP1 binds the 3′UTR of MICB at a GU-rich element and regulates its expression. (a) The predicted binding sequence of CUGBP1 at position 616-661 in the 3′UTR of MICB (top, bold black letters). Sequence of the mutation in the CUGBP1 predicted binding site, named GUmut (bottom). Mutated nucleotides are indicated in red. (b) RKO cells were transfected with one of two reporters: fused to the WT 3′UTR of MICB and to the GUmut 3′UTR. Forty-eight hours post transfection,Fireflyactivity was measured relative to theRenillaluciferase. Activity of the reporters was calculated relatively to the activity of the reporter fused to the WT 3′UTR. Shown is relative averaged mean±s.d. of combined three independent experiments. *P<0.002, by Student’st-test. (c) HEK293T cells were transduced with lentiviruses encoding MICB–CDS fused either to a MICB WT 3′UTR or to the GUmut 3′UTR. The cells were then transduced either with a specific shCUGBP1 shRNA (black histograms) or a control-shRNA (grey empty histograms). MICB (top) and MICA (bottom) expressions were evaluated by FACS. Filled grey histograms represent background staining. Data are a representative of four independent experiments. (d) Quantification of all FACS experiments performed in (c). Shown is the relative average MICB MFI±s.d. of all experiments. *P<0.02 by Student’st-test. (e) NK killing assay was performed on HEK293T cells transduced either with MICB–CDS fused to MICB WT 3′UTR or transduced with MICB–CDS fused to GUmut 3′UTR. These cells were then transduced either with a control-shRNA or with a specific shCUGBP1. Shown is relative average killing±s.d. of three independent experiments, calculated relative to the specific cells transduced with a control-shRNA. *P<0.005, by Student’st-test. Figure 8: CUGBP1 binds the 3′UTR of MICB at a GU-rich element and regulates its expression. ( a ) The predicted binding sequence of CUGBP1 at position 616-661 in the 3′UTR of MICB (top, bold black letters). Sequence of the mutation in the CUGBP1 predicted binding site, named GUmut (bottom). Mutated nucleotides are indicated in red. ( b ) RKO cells were transfected with one of two reporters: fused to the WT 3′UTR of MICB and to the GUmut 3′UTR. Forty-eight hours post transfection, Firefly activity was measured relative to the Renilla luciferase. Activity of the reporters was calculated relatively to the activity of the reporter fused to the WT 3′UTR. Shown is relative averaged mean±s.d. of combined three independent experiments. * P <0.002, by Student’s t -test. ( c ) HEK293T cells were transduced with lentiviruses encoding MICB–CDS fused either to a MICB WT 3′UTR or to the GUmut 3′UTR. The cells were then transduced either with a specific shCUGBP1 shRNA (black histograms) or a control-shRNA (grey empty histograms). MICB (top) and MICA (bottom) expressions were evaluated by FACS. Filled grey histograms represent background staining. Data are a representative of four independent experiments. ( d ) Quantification of all FACS experiments performed in ( c ). Shown is the relative average MICB MFI±s.d. of all experiments. * P <0.02 by Student’s t -test. ( e ) NK killing assay was performed on HEK293T cells transduced either with MICB–CDS fused to MICB WT 3′UTR or transduced with MICB–CDS fused to GUmut 3′UTR. These cells were then transduced either with a control-shRNA or with a specific shCUGBP1. Shown is relative average killing±s.d. of three independent experiments, calculated relative to the specific cells transduced with a control-shRNA. * P <0.005, by Student’s t -test. Full size image Next, to analyse whether CUGBP1 regulated the expression of MICB by binding to the above-mentioned GU-rich element, we generated two lentiviral constructs: (i) in which the MICB–CDS was fused to the WT 3′UTR of MICB, and (ii) in which the MICB–CDS was fused to the GUmut 3′UTR. HEK293T cells, which express very low protein levels of MICB ( Supplementary Fig. 6 ), were transduced with these two lentiviruses. Then, the cells were transduced with shRNAs: either with a Ctrl shRNA or with the specific shCUGBP1 and the levels of MICB were monitored by FACS. KD of CUGBP1 led to an increase in MICB expression only when it was expressed together with its WT 3′UTR ( Fig. 8c , top, left histogram). The change in MICB expression was statistically significant as quantified in Fig. 8d . In contract, no change in MICB expression was seen when MICB was expressed with the GUmut 3′UTR ( Fig. 8c , top, right histogram). In all cases, the levels of MICA were not affected ( Fig. 8c , bottom, quantified in Fig. 8d ). Finally, we performed NK killing assays on the above-mentioned HEK293T cells ( Fig. 8e ). In agreement with the FACS data ( Fig. 8c ), KD of CUGBP1 affected NK killing only when MICB was expressed with its WT 3′UTR and not when it was expressed with the GUmut 3′UTR. Thus, we concluded that CUGBP1 regulates the expression of MICB via the identified GU-rich element and affects NK-mediated killing. FUBP3 and HuR regulate MICB expression during DNA damage Finally, we wanted to investigate whether the RBP control of MICB expression also functions during cellular stress. We focused on the DNA-damage response as DNA damage is caused as a result of many insults (for example, exposure to ultraviolet light, viral infection and so on) and it was shown that MICB expression is induced during genotoxic stress [41] . We used the anthracycline drug Doxorubicin, which causes double-strand breaks and leads to the activation of the DNA-damage response. The stress was applied on primary human foreskin fibroblast (HFF) cells as tumour cell lines often suffer from genomic instability and thus might have an already active DNA-damage response. MICB expression was induced following doxorubicin treatment ( Supplementary Fig. 7 ) confirming previous findings [41] . Next, we transduced HFF cells with the various RBP-shRNAs and treated the cells with doxorubicin. Upon treatment, only the KD of FUBP3 and HuR, which are both known to play a role in the DNA-damage response [42] , [43] , resulted in an even greater increase in MICB expression as compared with Ctrl-shRNA-treated cells ( Fig. 9a , quantified in Fig. 9b ). In contrast, none of the RBP-shRNAs affected the levels of MICA ( Fig. 9a,b ). The levels of FUBP3 and HuR, in the KD HFF cell, before and following doxorubicin treatment were validated by WB ( Fig. 9c ). Finally, we performed NK killing assays on shCtrl, shFUBP3, shHuR and shSTAU2 (negative control)-transduced HFF cells following doxorubicin treatment and observed increased killing of the shFUBP3 and shHuR cells only ( Fig. 9d ). This demonstrates that FUBP3 and HuR regulate the expression of MICB under genotoxic stress in primary human cells. 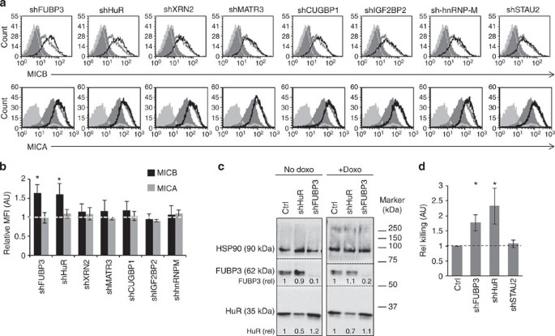Figure 9: FUBP3 and HuR regulate MICB expression during DNA damage. (a) FACS analysis of the expression of MICB (top) and MICA (bottom) on shRNA-transduced HFF cells prior (filled dark grey histogram) and following (empty grey/black histograms) doxorubicin treatment. The empty black histogram represents the specific shRNA-transduced HFF cells-treated cells (indicated above the histogram), the empty grey histogram represents control-shRNA-treated cells. The filled light grey histogram represents background staining. Data are representative of four independent experiments. (b) Quantification of all independent experiments performed in (a). Shown is the average MFI±s.d. relative to control-shRNA doxorubicin-treated HFF cells of all experiments. *P<0.005, by Student’st-test. (c) WB validation of FUBP3 and HuR–KD efficiency prior and following doxorubicin treatment (no Doxo and +Doxo, respectively). HSP90 served as a loading control. After blot transfer, the nitrocellulose membrane was cut, according to the molecular weight of HuR, FUBP3 and HSP90. Each membrane strip (borders indicated by the black dotted lines) was incubated with the respective primary antibody. (d) NK killing assay was performed on the indicated shRNA-transduced HFF cells (xaxis) following doxorubicin treatment. Shown is the relative average killing±s.d. of three independent experiments. Relative killing was calculated relative to the killing of control-shRNA-transduced HFF cells. *P<0.005 by Student’st-test. Figure 9: FUBP3 and HuR regulate MICB expression during DNA damage. ( a ) FACS analysis of the expression of MICB (top) and MICA (bottom) on shRNA-transduced HFF cells prior (filled dark grey histogram) and following (empty grey/black histograms) doxorubicin treatment. The empty black histogram represents the specific shRNA-transduced HFF cells-treated cells (indicated above the histogram), the empty grey histogram represents control-shRNA-treated cells. The filled light grey histogram represents background staining. Data are representative of four independent experiments. ( b ) Quantification of all independent experiments performed in ( a ). Shown is the average MFI±s.d. relative to control-shRNA doxorubicin-treated HFF cells of all experiments. * P <0.005, by Student’s t -test. ( c ) WB validation of FUBP3 and HuR–KD efficiency prior and following doxorubicin treatment (no Doxo and +Doxo, respectively). HSP90 served as a loading control. After blot transfer, the nitrocellulose membrane was cut, according to the molecular weight of HuR, FUBP3 and HSP90. Each membrane strip (borders indicated by the black dotted lines) was incubated with the respective primary antibody. ( d ) NK killing assay was performed on the indicated shRNA-transduced HFF cells ( x axis) following doxorubicin treatment. Shown is the relative average killing±s.d. of three independent experiments. Relative killing was calculated relative to the killing of control-shRNA-transduced HFF cells. * P <0.005 by Student’s t -test. Full size image It is still unknown why humans encode eight different stress-induced NKG2D ligands and how these ligands are regulated. A possible answer to the first question might be that such a variety of NKG2D ligands make it difficult for a pathogen or a tumour to develop mechanisms to interfere with the transmission of stress and/or danger signals. Another possible explanation (which does not contradict the first explanation) is that the stress-induced ligands are differentially regulated and are therefore differentially induced upon different stresses and conditions. The results presented here support the later hypothesis as we demonstrate that even though MICB and MICA share more than 80% similarity in their amino-acid sequence they are post transcriptionally differentially regulated by RBPs. To identify RBPs that interact with MICA and/or MICB, we utilized an RNA-AP method and identified six RBPs that bind to the 3′UTR of MICB (but not the 3′UTR of MICA) and regulate its expression. Gene expression is regulated both by nuclear and cytoplasmic RBPs, and while nuclear RBPs mainly control transcription and RNA processing, cytoplasmic RBPs control localization, stability and translation of the transcript. We focused on cytoplasmic RBPs by using cytoplasmic extracts while excluding nuclear proteins. Thus, our study was designed to identify predominantly RBPs affecting mRNA stability, turnover and translation. It is likely that additional nuclear (or cytoplasmic) RBPs exist that bind to MICB mRNA and control its intracellular fate. We used RIP experiments to demonstrate that all of the identified RBPs, except MART3, which we were unable to precipitate, directly interact with MICB, but not with MICA transcripts in living cells. Of note, in the WB validation of RIP assay, although the prominent band was of the precipitated RBP, additional proteins bands were detected suggesting that other proteins were precipitated as well. Thus, it is possible that these additional proteins were those that bind MICB and that the identified RBPs regulated MICB indirectly. Yet, this scenario is highly unlikely, as we have demonstrated the effect of the RBPs on MICB expression by various modalities that includes over expression, KD of the various RBPs and when possible, mutation. Our approach identified six novel MICB regulators; five negative regulators: FUBP3, HuR, XRN2, MATR3 and CUGBP1; as well as one positive regulator, IGF2BP2-short. The MICB-regulating RBPs identified in the current study include well-known RBPs with already established roles in well-known pathologies functioning as regulators of additional genes; HuR in cancer, metastasis and angiogenesis [44] , CUGBP1 in muscle pathologies [45] , [46] and liver dysfunction [29] and IGF2BP2 is implicated in the aetiology of late onset of type-2 diabetes [47] . Importantly, while regulating the expression of MICB, the identified RBPs did not affect MICA expression. They were not precipitated with the MICA 3′UTR and binding sequences of these RBPs are absent from the 3′UTR of MICA (except one single AU-rich sequence, Supplementary Fig. 5 ). Furthermore, none of the assays employed in this manuscript including KD, overexpression or RIP indicated that these RBPs can affect MICA expression. The fact that sequence-specific RBPs were precipitated only with the 3′UTR of MICB and not with MICA was surprising because MICA and MICB are commonly regulated by similar mechanisms. For example, although MICA has a much shorter 3′UTR than MICB (174 bp versus 1231, bp, respectively), most of the identified cellular miRNAs that target the 3′UTR of MICB target the MICA 3′UTR, as well (miR-17, -20a, -93, -106b, -372, -373 and -520d) [18] . Whether an RBP will negatively or positively regulate a specific transcript is difficult to predict. Moreover, the determinants needed for the RBP-mediated control and the details of the mechanisms by which RBPs regulate gene expression are virtually unknown. When we analysed the sequence of the control UTR used in the RNA-AP for MICB (the 3′UTR of CASQ2), we found one AU-rich element, several MATR3-binding sequences and multiple IGF2BP2-binding sequences ( Supplementary Fig. 8 ), and yet the identified RBPs did not bind to the 3′UTR of CASQ2 ( Fig. 1 ). These results indicate that we are far from a complete understanding about the mode of binding of the RBPs. This also emphasizes the importance of conducting precipitation experiments, followed by validation experiments to identify genuine mRNA–RBPs interactions. RBPs are known to interact not only with additional RBPs but also with miRNA-bearing complexes [48] . Indeed, as expected, RNA-induced silencing complex subunits were identified in the MS analysis that we performed. These interactions can be quite complex as RBPs can either interact in a competitive manner or in synergism with the miRNAs that also regulate the expression of the specific transcript [48] . Interestingly, of the ten cellular miRNAs that are known to regulate MICB [18] , [19] , [20] , only one miRNA, miR-10b, was found to overlap with an RBP consensus sequence ( Supplementary Fig. 9a ), and none of the herpesviruses’ miRNAs [49] , [50] , which we characterized previously to regulate MICB, overlapped with an RBP sequence ( Supplementary Fig. 9b ). These observations suggest that the cellular miRNAs that target MICB [18] , [19] , [20] and in particular, the herpes virus miRNAs [49] , [50] might have evolved to bind the 3′UTR at sites that are not occupied by RBPs. It will be interesting to investigate in the future the protein–protein interactions between the different RBPs and the protein–miRNA interaction and their relations to the control the expression of MICB. Danger is sensed by the immune system via stress molecules such as MICB to activate NK cells that quickly eradicate the hazardous cell. Thus, we were curious to test whether the RBP-mediated regulation of MICB also functions during stress. DNA damage occurs constantly; by exposure to ultraviolet light, by replication cycles and proliferation, by respiration and metabolic processes, by cell transformation or by viral infections. Nonetheless, it is still a mystery how DNA damage translates to the upregulation of the stress-induced ligands. Although it was previously demonstrated that DNA damage induces MICB expression, the exact mechanism is still unknown. Moreover, DNA damage increases the relative abundance of the MICB transcript, but it is unknown whether this is due to de novo transcription or due to a change in mRNA stability. Here we demonstrate that FUBP3 and HuR, which are phosphorylated by DNA damage-activated kinases [42] , [43] , control the stability of the MICB transcript and negatively regulate MICB during genotoxic stress. Interestingly, the expression of MICB is not induced following KD of FUBP3 and HuR in untreated HFF cells ( Supplementary Fig. 10 ), while it is induced in RKO cells ( Fig. 2b ). This suggests that in healthy cells under normal conditions, the regulation of MICB is very strict and less permissive than in cancer cells. It might be that under normal conditions, the expression of the stress-induced ligands should be induced only after intolerable stress to the cell, to prevent excessive and unwanted damage. In contrast, tumour cells such as RKO cells frequently suffer from genomic instability, which is a potent inducer of NKG2D ligands. Thus, tumour cells might have lost some regulatory breaks that prevent the expression of the NKG2D ligands. The recognition of the stress-induced ligands by NKG2D is one of the best examples of how danger is recognized by the immune system. We demonstrate here a novel mode of regulation of MICB, a stress-induced ligand, by RBPs. Our discovery of the first six RBPs that control MICB expression might open the door for the discovery of new control mechanisms governing immunosurveillance by NK cells. This might lead to the development of new therapeutics and new avenues of research elucidating the mechanisms by which the NKG2D ligands are induced during tumor transformation, virus infection, genotoxic stress and autoimmunity. Generation of pBSII-UTR plasmids The 3′UTRs of MICA (sense and antisense orientation), MICB (sense and antisense orientation), TAF6 (a control 3′UTR for MICA) and CASQ2 (a control 3′UTR for MICB) were cloned into the pBSII plasmid using the primers listed in Supplementary Table1 . Prior to in vitro transcription, the plasmids were linearized with the SalI restriction enzyme. In vitro transcription and RNA labelling In vitro transcription was performed with the Megascript T7 in vitro transcription kit (Ambion) in the presence of Biotin-16-UTP (GE Healthcare) according to the manufacturer’s instructions with modifications [27] . RNA-AP The assay was essentially performed as described previously [27] . Briefly, HEK293T and RKO cells were grown to 90% confluence in DMEM media with 10% fetal calf serum. Cells were washed twice with 1 × PBS, scraped off the plates in 10 ml of 1 × PBS and collected at 4 °C in the cold room. Cells were spun down at 1,900 g , 4 °C for 10 min. Pellets were combined, washed in PBS and used for cytoplasmic extraction by hypotonic buffer. Protein concentrations were determined by BCA assay and 1 mg of protein was used for each cell line for every lane. Streptavidin beads (GE Healthcare) were blocked with yeast tRNA (Sigma), and mixed with the various RNA molecules for overnight incubation at 4 °C. Proteins were eluted with 6 M urea, 0.01% NP40, 1 mM DTT, precipitated and then run on an SDS–PAGE protein gel. Antibodies for flow cytometry and WB The anti-hMICA (159227, 0.2 μg per 100,000 cells) anti-hMICB (236511, 0.2 μg per 100,000 cells) antibodies were purchased from R&D systems. In all FACS experiments, the anti-mouse-DyLight649 secondary antibody was used (Jackson ImmunoResearch, final dilution 1:500). For WB, the following antibodies were used: anti-FUBP3 (ab108222, final dilution 1:500), anti-HuR (03-102, Millipore, final dilution 1:10,000), anti-IGF2BP2 (03-251, Millipore, final dilution 1:10,000), anti-XRN2 (H-30, sc-99237, Santa Cruz, final dilution 1:500), anti-MATR3 (AV0923, Sigma-Aldrich, final dilution 1:500), anti-CUGBP1 (03-104, Millipore, final dilution 1:10,000), anti-hnRNP-M1-4 (03-100, Millipore, final dilution 1:10,000), anti-c-JUN (06-225, Millipore), final dilution 1:10,000, anti-HSP90 (05-594, Millipore, final dilution 1:10,000) and anti-alphaTubulin (AA13, Sigma-Aldrich, final dilution 1:1000). Generation of lentiviral constructs The various RBP–KD vectors and control vector were present in the pLKO.1-puro plasmids and were purchased from Sigma-Aldrich. HEK293T and RKO cells were grown in the presence of 2.5 μg ml −1 puromycin for selecting the positive cells. Cloning of the various RBPs was performed into the pHAGE.CMV.IRES.eGFP plasmid. Cloning of MICB–CDS fused either to the WT 3′UTR or the GUmut 3′UTR was performed into the EF.CMV.RFP lentiviral vector, purchased from Addgene (plasmid #17619). Generation of lentiviruses was achieved according to the manufacturer’s instructions. The specific primers sequences are listed in Supplementary Table 2 . RNA extraction and cDNA preparation Total RNA was extracted with TRI reagent (Sigma), and was treated with Turbo -DNase (Ambion), and a poly(A) tail was added using the poly(A) kit (Ambion). For generation of cDNA libraries, the M-MLV reverse transcriptase (Invitrogen) was used for reverse transcription (according to the manufacturer’s instructions), in the presence of an adaptor primer. Detection of the various transcripts was performed with the primers listed in Supplementary Table 3 . Luciferase reporter assay The 3′UTR of MICB was cloned downstream to a Firefly reporter into the pGL3 vector (Promega) as described [49] . To generate the partial UTR reporters, the full UTR was cut with XbaI and the two fragments were cloned into the pGL3 plasmid. Twenty-four hours prior to transfection of the reporter plasmids, cells were plated to 50% confluence in 24-well plates in triplicates. A quantity of 200 ng per well of the pGL3 vector and 50 ng per well of the pRL-CMV vector were transfected with the TransIT-LT1 transfection reagent (Mirus Biotech), and relative Firefly activity was assessed 48 h post transfection. Firefly/Renilla activity ratio was normalized to that in the control cells, and then the relative activity of the reporter was calculated. NK cell cytotoxicity assays The study was approved by the Hadassah Medical Center Institutional Review Board and was performed according to the Declaration of Helsinki, good clinical practice guidelines and the human experimentation guidelines of the Israeli Ministry of Health. All donors gave written informed consent. NK cells were isolated from healthy donors via MACS separation (Miltenyi Biotech) and grown in the presence of IL-2 (Peprotech). Target cells were grown over night in the presence of [ 35 S]Methionine added to a Methionine-free media (Sigma). Before incubation with the effectors, cells were washed, counted and 5,000 cells per well were plated. For each target, the spontaneous [ 35 S]release was calculated by cells, which were not incubated with effector cells, and maximum [ 35 S]-release was calculated by applying 100 μl 0.1 M NaOH to the target cells. The level of [ 35 S]-release was measured after 5 h of incubation with effectors (at 37 °C) by a β-counter TopCount (Packard). Doxorubicin treatment Doxorubicin was purchased from Sigma-Aldrich (cat. d1515). Twenty-four hours prior to stress induction, cells were plated to 80% confluence. A volume of 2 μg ml −1 doxorubicin was applied to the growing media for 2 h. After 2 h, the media was removed, cells were washed and new media was added. After 48 h, the levels of MICB were analysed by FACS. ActD treatment ActD was purchased from Sigma-Aldrich (cat. A9415). Twenty-four hours prior to treatment induction, cells were plated to 80% confluence. A volume of 5 μg ml −1 ActD was applied to the growing media for 16 h. Then, total RNA was isolated, DNase treated, reversed transcribed and qRT–PCR analysis was performed. RNA Immunoprecipitation The assay was performed as described [34] . Briefly, RNA was purified using TRI reagent (T9424, Sigma-Aldrich), and the Protein A/G PLUS-Agarose beads (sc-2003, Santa Cruz) were used. RKO cells were used for the validation of the RBP–MICB–mRNA interactions. Total cell lysate was prepared using an ice cold lysis buffer, then the lysate was precleared using Protein A/G PLUS-Agarose beads. Then the cleared lysate was incubated at 4 °C overnight with each specific antibody or immunoglobulin Control. Agarose beads were then added for an additional 4 h. After several washing cycles, RNA was isolated using the TRI reagent and the presence of the MICB and MICA transcripts was detected via qRT–PCR. The following antibodies were used: anti-FUBP3 (ab108222), anti-HuR (03-102, Millipore), anti-IGF2BP2 (03-251, Millipore), anti-XRN2 (H-30, sc-99237), anti-CUGBP1 (03-104, Millipore), anti-hnRNP-M1-4 (03-100, Millipore). Enrichment was evaluated by qRT–PCR and was calculated relative to the levels of the specific transcript in the total input samples, by . How to cite this article : Nachmani, D. et al . RNA-binding proteins regulate the expression of the immune activating ligand MICB. Nat. Commun. 5:4186 doi: 10.1038/ncomms5186 (2014).